The non-canonical poly(A) polymeraseFAM46Cacts as an onco-suppressor in multiple myeloma FAM46C is one of the most frequently mutated genes in multiple myeloma. Here, using a combination of in vitro and in vivo approaches, we demonstrate that FAM46C encodes an active non-canonical poly(A) polymerase which enhances mRNA stability and gene expression. Reintroduction of active FAM46C into multiple myeloma cell lines, but not its catalytically-inactive mutant, leads to broad polyadenylation and stabilization of mRNAs strongly enriched with those encoding endoplasmic reticulum-targeted proteins and induces cell death. Moreover, silencing of FAM46C in multiple myeloma cells expressing WT protein enhance cell proliferation. Finally, using a FAM46C-FLAG knock-in mouse strain, we show that the FAM46C protein is strongly induced during activation of primary splenocytes and that B lymphocytes isolated from newly generated FAM46C KO mice proliferate faster than those isolated from their WT littermates. Concluding, our data clearly indicate that FAM46C works as an onco-suppressor, with the specificity for B-lymphocyte lineage from which multiple myeloma originates. Mass sequencing of cancer genomes has revealed genomic landscapes of human cancers allowing for the identification of a large number of potential tumor suppressors and oncogenes. FAM46C , a gene whose physiological function was largely unknown, is one of the most frequently mutated genes in multiple myeloma (MM), following the well-known proto-oncogenes, KRAS , NRAS , and BRAF [1] , [2] . Deletions of FAM46C gene 1p12 locus (del(1p)) have been found in ~20% of MM cases and are associated with short progression-free survival and decreased overall survival [3] , [4] . Except of chromosomal aberrations, recurrent homozygotic or hemizygotic somatic point mutations have been identified in about 10% of MM cases, depending on studies based on whole-genome- or whole-exome sequencing [3] , [5] , [6] , [7] , [8] . To date, more than 70 unique somatic mutations across whole FAM46C gene sequence have been identified, many of which are frameshift or nonsense mutations ( https://research.themmrf.org ) [1] . Importantly, FAM46C mutations are specific to MM since no other cancer type with statistical significant enriched in FAM46C mutations has been described so far [9] . The high frequency of mutation in the FAM46C gene allowed it to be classified as MM driver-gene, which may function as a tumor suppressor even though it does not contain mutational hotspots [6] , [10] , [11] . FAM46C mutations are also frequently found in stable human myeloma cell lines. In addition, FAM46C has been identified as a type I interferon-stimulated gene, overexpression of which slightly enhances replication of some viruses [12] , [13] . FAM46C belongs to a FAM46 metazoan-specific family of proteins, which has 4 members in humans that are very similar at the protein level with a degree of sequence identity of at least 56.9%. There is currently very little functional data on FAM46 proteins. Positional cloning in mouse revealed that mutations in FAM46C gene cause anemia [14] . The only publication about this phenomenon is the PhD thesis of Tian [14] . The author performed initial biochemical characterization of FAM46C and concluded that it is a RNA-binding protein that stabilizes specific mRNAs in reticulocytes, including that of alfa-globin, which correlates with poly(A) tail shortening. Recent bioinformatic fold recognition searches classified FAM46C as a member of the novel nucleotidyltransferases (NTases) family; however, this study did not provide reliable predictions of molecular function [15] , [16] . NTases transfer nucleoside monophosphate (NMP) from nucleoside triphosphate (NTP) to an acceptor hydroxyl group and are involved in many biological processes, including mRNA polyadenylation and editing, DNA repair and chromatin remodeling, intracellular signal transduction, and regulation of protein activity [15] , [17] . Here we performed the first comprehensive molecular characterization of FAM46C . We show that FAM46C is an active poly(A) polymerase that positively regulates expression of ER-targeted mRNAs. Furthermore, the presented data strongly indicate that FAM46C is a B-cell lineage-specific growth suppressor as silencing of FAM46C in MM cells that express the wild-type protein enhances cell division, whereas introduction of wild-type FAM46C into MM that express the protein with mutations leads to growth arrest; also, primary B cells isolated from FAM46C KO animals proliferate faster. Thus, we describe FAM46C as an onco-suppressor non-canonical poly(A) polymerase. FAM46C encodes a poly(A) polymerase that enhances gene expression The FAM46 family of proteins exists only in animals. In vertebrates, all its members have the same architecture. They contain domains that are very distantly related to the catalytic and associated domains of poly(A) polymerases, and they lack any detectable RNA-binding domains [15] . The putative catalytic residues of FAM46C are preserved, indicating that this protein may indeed be an active poly(A) or poly(U) polymerase (Supplementary Fig. 1 ). In order to confirm predicted molecular activity, we purified recombinant FAM46C and its mutant version, in which acidic residues of the putative catalytic center, expected to coordinate divalent cations, were replaced by alanines (D90A and D92A; FAM46C mut ). This was followed by an in vitro polyadenylation assay using a A 15 oligoribonucleotide RNA as a substrate. Wild type, but not catalytic mutant, protein was able to extend the RNA substrate in vitro in the presence of ATP and divalent metal ions (Mn 2+ ) (Fig. 1a, b ), indicating that FAM46C is a poly(A) polymerase. However, due to the relatively low activity of recombinant FAM46C (likely related to its intrinsic low solubility and aggregation), we validated the result using recombinant FAM46D, which was more soluble; the sequences of the two proteins are highly similar (Supplementary Fig. 1 ). FAM46D displayed poly(A) polymerase activity and was able to extend A 15 oligoribonucleotide substrate; its activity was significantly higher compared to that of FAM46C (Fig. 1c ). Fig. 1 FAM46C interacts with RNA and is an active RNA poly(A) polymerase in vitro and in vivo. a Recombinant FAM46C WT (lanes 8–13), but not its catalytic mutant FAM46C mut (lanes 2–7), displays poly(A) polymerase activity in vitro. Reaction products (using 32 P-labeled (A) 15 as substrate) were separated in denaturing PAGE gels and visualized by autoradiography. b SDS-PAGE analysis of recombinant FAM46C WT and its catalytic mutant FAM46C mut . c FAM46D WT is an active poly(A) polymerase in vitro and requires Mn 2+ ions for its activity. Purified protein was incubated with 32 P-labeled (A) 15 primer in the presence of ATP and divalent cations as follows: Mg 2+ (lanes 4–6), both Mg 2+ /Mn 2+ (lanes 7–9), or Mn 2+ (lanes 10–12). Control reactions were carried out without the protein (lanes 1–3). d FAM46C interacts with RNA in human cells. Autoradiography of UV cross-linked 32 P-labeled RNAs co-purified with FAM46C WT GFP from HEK293 cells stably expressing the fusion protein (lanes 3–4) and from control empty cells (lanes 1–2). Immunoprecipitated RNA-protein complexes were separated by SDS-PAGE, transferred to nitrocellulose membrane, stained with Ponceau S, and subsequently autoradiographed. The right panel shows the Ponceau S stained blot merged with autoradiogram Full size image In order to determine the molecular function of FAM46C, we evaluated whether this protein could interact with RNA at the cellular level. Stable HEK293 cells expressing FAM46C WT -GFP were UV cross-linked and the tagged proteins were immunoprecipitated using anti-GFP antibodies. Co-purified RNA was visualized by 32 P-labeling of RNA-protein covalent crosslinks. Strong enrichment of RNA was observed in cross-linked, FAM46C-positive samples compared to control cells and non-crosslinked samples (Fig. 1d ), demonstrating that FAM46C binds to RNA and may act as an RNA poly(A) polymerase in human cells. Non-canonical poly(A) polymerases may enhance overall gene expression by extending the poly(A) tails of dormant messenger RNAs (like GLD2) in the cytoplasm or trigger rapid exosome-mediated RNA decay by oligoadenylation of target RNA in the nucleus (as in the case of TRF4) [18] . In order to examine intracellular localization of the FAM46C protein, HEK293T, RPMI826 (MM), H929 (MM), SKMM1 (MM), HL60 (promyelocytic leukemia) and Raji (B-cell lymphoma) cell lines were transduced with constructs encoding the FAM46C WT -GFP fusion gene. Confocal microscopy revealed simultaneous nuclear and cytoplasmic localization of FAM46C in all tested cell lines, as expected for non-canonical poly(A) polymerases (Fig. 2 ), demonstrating the possibility of both RNA stabilizing and destabilizing functions. Fig. 2 FAM46C shows both nuclear and cytoplasmic localization. HEK293T, RPMI826 (MM), H929 (MM), SKMM1 (MM), HL60 (promyelocytic leukemia) and Raji (B-cell lymphoma) cell lines were transduced with constructs encoding the FAM46C WT –GFP fusion gene. Non-transduced cells were used as a control. Fluorescence images for GFP and Hoechst nucleic acid stain, as well as merged images, are shown. Scales bars (10 µm) are shown for each set of images Full size image To further analyze FAM46C function in cells, we performed an RNA-tethering assay. HEK293 cells were co-transfected with a construct expressing Renilla luciferase (RL) containing five boxB sites in its 3′-UTR, Firefly luciferase (FL) control reporter and FAM46C WT harboring the N-terminal λN boxB-binding domain and HA-tag [19] . After 24 h, the levels of reporter protein were analyzed, which revealed that tethering a wild-type FAM46C enhances expression of RL more than 7-fold ( Fig. 3a, d ) . Several additional controls were applied to prove that the catalytic activity of FAM46C was indeed responsible for the enhanced expression of RL reporter: (1) tethering of the catalytic FAM46C mutant had little effect on RL reporter expression ( Fig. 3a, d ) ; (2) a RL reporter with a cyclic phosphate at the 3′-end generated by a hammerhead ribozyme, which cannot be polyadenylated, was insensitive to FAM46C tethering ( Fig. 3b, d ) ; (3) expression of FAM46C without the λN domains did not enhanced expression of the reporter ( Fig. 3c, d ) . At the RNA level, northern blot analysis revealed that enhanced expression of RL upon FAM46C WT tethering correlated with increased steady state levels and slower migration of its mRNA ( Fig. 3e, f ) . This was not observed for the RL reporter with a cyclic phosphate at the 3′ ( Fig. 3e, f ) . Quantifications of control FL reporter mRNA revealed no effect of FAM46C on its expression (Fig. 3g ). Furthermore, northern blot analysis of poly(A) enriched-RNA fractions revealed significant increases in steady-state levels and slower migration of RL mRNA in samples where FAM46C WT was tethered (Fig. 3h ). Next, we confirmed that the observed RL mRNA lengthening is indeed caused by polyadenylation of mRNA 3′-end using an RNase H cleavage assay with oligo(dT) 25 (Fig. 3i ). In addition, RNA from cells after FAM46C was tethered to RL mRNA was fractionated based on the lengths of poly(A) tails using oligo dT sepharose resin. Northern blot analysis revealed that more RL mRNA molecules were present in fractions with longer poly(A) tails, confirming that it is polyadenylated by FAM46C (Supplementary Fig. 2a ). The same effect was observed for FAM46D indicating that they have similar properties (Supplementary Fig. 2b ). Fig. 3 FAM46C tethering leads to polyadenylation and enhanced expression of a Renilla luciferase (RL) reporter. Analysis at the protein level ( a – d ): a FAM46C tethering increases RL reporter protein levels. HEK293 cells were co-transfected with a construct expressing RL, containing five boxB sites in its 3′-UTR, Firefly luciferase (FL) control reporter and FAM46C WT harboring the N-terminal λN boxB-binding domain and HA-tag. Western blot detection of RL in mock-transfected cells (lane 1) and after NHA-FAM46C WT (lane 2) or NHA-FAM46C mut (lane 3) tethering. Expression of NHA-tagged FAM46C proteins were confirmed using an α-HA antibody. DBC1 served as a loading control. Asterisks indicate cross-hybridization signals. b Expression of RL5boxHSL + HhR reporter with a cyclic phosphate at the 3′ end generated by a hammerhead ribozyme was not enhanced upon FAM46C tethering. The experiment was performed as in a . c Expression of the FAM46C without λN domains did not enhance expression of the reporter. The experiment was performed as in a . d Quantifications of RL protein normalized by the internal FL reporter related to experiments from a – c . RNA analysis ( e – i ): e northern blot detection of RL mRNA using total RNA from HEK293 cells after tethering of NHA-FAM46C WT or NHA-FAM46C mut to RL5box (lanes 1–3) or RL5boxHSL + HhR with a cyclic phosphate at the 3′ end (lanes 4–6). f Quantifications of RL mRNA. g RT-qPCR analysis of the FL control reporter. h Northern blot detection of Renilla luciferase using poly(A) + fraction from HEK293 cells after tethering of NHA-FAM46C WT or NHA-FAM46C mut ( i ) Poly(A) tails added to reporter mRNA can be removed by RNase H treatment in the presence of oligo(dT) 25 . High-resolution northern blot analysis of RL mRNA from control HEK293 cells (lanes 1–2), after tethering of NHA-FAM46C WT (lanes 3–4) or NHA-FAM46C mut (lanes 5–6). The data in d , f , g are shown as a mean value ± SD ( n = 3) Full size image In order to determine whether the observed increase in reporter expression was due to mRNA stability, we evaluated the half-life of RL mRNA. Cells were transfected with pRL-5BoxB and pNHAFAM46C WT or pNHAFAM46C mut . After 24 h, transcription was inhibited for 4, 8, and 12 h by the addition of actinomycin D. Northern blot, followed by densitometry quantifications analyses of steady state levels of RL mRNA obtained from appropriate time points, revealed significant increases in the mRNA half-life of the molecules polyadenylated by FAM46C compared to control cells (Supplementary Fig. 2c, d ). Therefore, it was concluded that FAM46C is an active poly(A) polymerase which, when tethered, stabilizes mRNA and enhances gene expression. 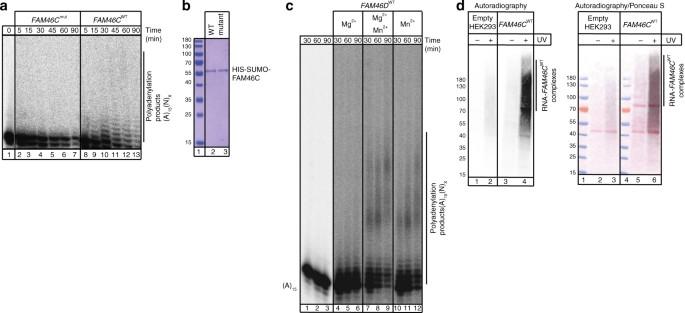Fig. 1 FAM46C interacts with RNA and is an active RNA poly(A) polymerase in vitro and in vivo.aRecombinant FAM46CWT(lanes 8–13), but not its catalytic mutant FAM46Cmut(lanes 2–7), displays poly(A) polymerase activity in vitro. Reaction products (using32P-labeled (A)15as substrate) were separated in denaturing PAGE gels and visualized by autoradiography.bSDS-PAGE analysis of recombinant FAM46CWTand its catalytic mutant FAM46Cmut.cFAM46DWTis an active poly(A) polymerase in vitro and requires Mn2+ions for its activity. Purified protein was incubated with32P-labeled (A)15primer in the presence of ATP and divalent cations as follows: Mg2+(lanes 4–6), both Mg2+/Mn2+(lanes 7–9), or Mn2+(lanes 10–12). Control reactions were carried out without the protein (lanes 1–3).dFAM46C interacts with RNA in human cells. Autoradiography of UV cross-linked32P-labeled RNAs co-purified with FAM46CWTGFP from HEK293 cells stably expressing the fusion protein (lanes 3–4) and from control empty cells (lanes 1–2). Immunoprecipitated RNA-protein complexes were separated by SDS-PAGE, transferred to nitrocellulose membrane, stained with Ponceau S, and subsequently autoradiographed. Therightpanel shows the Ponceau S stained blot merged with autoradiogram FAM46C is an MM cell growth suppressor To study FAM46C in the context of MM pathogenesis, we took advantage of the established MM cell lines, some of which harbor early frameshift mutations in FAM46C : SKMM1 (Homozygous p.I173fsX36) and H929 (hemizygous p.L93fsX15) (Supplementary Table 1 ). In order to reintroduce wild-type FAM46C into these cell lines, we designed a lentiviral vector allowing for the expression of C-terminally GFP-tagged protein under the control of the spleen focus-forming virus (SFFV) promoter, which is active in hematopoietic cells [20] . Initially, we evaluated transduction efficiency and protein expression levels using control HEK293T cells, which were transduced with lentiviruses carrying FAM46C WT -GFP, FAM46C mut -GFP, or GFP as control, using different multiplicities of infection (MOIs; from 1 to 4). In all cases, stable cell lines were obtained with >95% efficiency as verified by flow cytometry for GFP-expressing living cells (Supplementary Fig. 3a ). No significant growth phenotypes were observed in HEK293T cells. A cytometric analysis of the cell cycle revealed higher number of cells in the G0/G1 phase; however, this observation could be a side effect associated with lentiviral particles, as it was not correlated with the activity of the FAM46C protein. Next, we transduced SKMM1, H929 (both mutated in the endogenous FAM46C locus), and RPMI8226 (with wild-type FAM46C sequence) with lentiviruses carrying FAM46C WT -GFP, FAM46C mut -GFP, and GFP constructs at MOIs from 1 to 4. Cytometric analysis of cell cultures was used to monitor the effect of FAM46C expression up to 11 days post transduction. Three days after transgene delivery, most of the tested cell lines expressing FAM46C WT had reduced growth rate and increased number of dead cells (Fig. 4a, b ); this effect was positively correlated with high FAM46C WT virus titer levels (Supplementary Fig. 4b ). Interestingly, in SKMM1 cells, the cytostatic effect of FAM46C WT expression was observed later in comparison to H929 or RPMI8226 cells and was best visible from the ninth day after transduction. Cytostatic effect was also observed for constructs with other tags at the N and C termini of FAM46C protein (FLAG-FAM46C WT , FAM46C WT -FLAG, GFP-FAM46C WT , and NHA-FAM46C WT ; Supplementary Fig. 4 ). We also tested other MM cell lines (MM1.S, MM1.R) and observed the same effects. Importantly, in contrast to FAM46C WT -GFP, expression of FAM46C mut -GFP or GFP only, did not cause cell death and stable MM cell lines were established (Fig. 4a, b ). This observation indicate that cytotoxic and cytostatic effects of FAM46C overexpression depend on its enzymatic activity. Moreover, overexpression of GFP-tagged nucleotidyltransferases such as canonical (PAPOLA) or non-canonical poly(A) polymerases (POLS or GLD2) in SKMM1 cell lines did not cause strong cytostatic effects (Supplementary Fig. 5 ), since the toxicity was visible only at early time points post transduction and stable cell lines were derived. This suggests a unique influence of FAM46C on MM cell viability. Fig. 4 FAM46C control survival and proliferation of multiple myeloma cells. a – c Expression of FAM46C WT induces death in multiple myeloma cells. a An example gating strategy for defining transduction efficiency and cell viability. Forward scatter (FSC) and side scatter (SSC) gate were used to separate debris from intact cells. Viability of RPMI8226 cells overexpressing either FAM46C WT -GFP or FAM46C mut -GFP was analyzed using propidium iodide (PI) staining on the 11th day post-transduction. GFP expression (GFP+) was evaluated in parallel in PI-negative cells. b , c Summary of flow cytometry analyses presented as bar graphs showing GFP expression level and reduced viability of multiple myeloma cell lines (SKMM1, H929, and RPMI8226 in b and Raji and HL60 in c throughout the time course of GFP, FAM46C WT -GFP, and FAM46C mut -GFP expression. The data are presented as percentage of cells ± SD ( n = 3). P values were calculated using two-way ANOVA tests (* P < 0.05, ** P < 0.01, *** P < 0.001, **** P < 0.0001). d , e shRNA-mediated silencing of FAM46C enhances proliferation rate of RPMI8226 MM cell line expressing wild-type protein but not SKMM1 harboring FAM46C mutation. Cells were transduced with lentiviral vectors expressing shRNA and empty vector as control. Stable transduced cell lines were stained with CFSE. Cell division was monitored by flow cytometry after 48 and 72 h by levels of CFSE dilution. d Reverse transcription qPCR analysis of the FAM46C silencing efficiency. Bars represent mean values ± SD ( n = 3). e The rate of proliferation of shRNA treated cells normalized to the control transduction. Bars represent mean values ± SD. P -values were calculated using Student’s t -test (* P < 0.05), ( n = 3) Full size image Finally, in order to determine if FAM46C toxicity is restricted to MM cells, other hematological cell lines, including HL60 (promyelocytic leukemia) and Raji (B-cell lymphoma), were transduced with lentiviruses carrying FAM46C WT -GFP, FAM46C mut -GFP, and GFP. Unlike in MM cells, expression of FAM46C had no effect on HL60 or Raji cell growth and viability, and these lines were established after cell sorting (Fig. 4c ). It was concluded that FAM46C expression specifically induces cell death of MM cells, however, we cannot exclude that reduced toxicity of FAM46C for HL60 and Raji cell is not related to lower expression levels of the transgene. Furthermore, in order to verify if FAM46C may positively regulate gene expression in MM cells we have conducted tethering assays performed similarly to the one described for HEK293 cells but implemented for SKMM1 and H929 cells. As expected, tethering of FAM46C WT but not FAM46C mut in MM cell lines enhanced the expression of the reporter mRNA (Supplementary Fig. 6 ). Mutations in FAM46C are found only in a fraction of MM cases. In order to check whether the effect of FAM46C on cell survival and proliferation is general to MM cells, we silenced FAM46C expression in RPMI8226, a MM cell line expressing wild-type FAM46C . To this end, we derived stable cell lines transduced with lentiviral vectors expressing three different shRNA targeting FAM46C . Although the level of silencing was moderate (~ 50%, Fig. 4d ), basically all shRNAs led to an moderately increased proliferation rate of RPMI8226 cell line as measured using CFSE cell tracer (Fig. 4e ). Such an effect was not observed in the SKMM1 MM cell line harboring FAM46C mutations (Fig. 4e ). This result strongly suggests that FAM46C suppresses the growth of all MM cells. FAM46C KO enhances B lymphocyte proliferation rate The analysis of MM cell lines revealed that FAM46C expression affects their growth and survival. Our intensive trials to raise or purchase specific antibodies that recognized FAM46C failed and so we were unable to verify endogenous FAM46C levels in MM cells. Thus, to study the expression of FAM46C in the B-cell lineage, from which MM originates, we have generated a FAM46C-FLAG knock-in mouse using CRISPR/Cas9 methodology. The animals did not display any detectable phenotypes. We have used western blot analysis of IL4 and LPS activated splenocytes and found that FAM46C expression was very strongly enhanced upon activation (Fig. 5a ). Furthermore, cell fractionation experiments revealed that it is localized mainly in the cytoplasm (Fig. 5b ), which is generally in agreement with our localization studies based on confocal imaging. Such result suggests that FAM46C may act as a non-canonical poly(A) polymerase in the B lymphocyte lineage. Fig. 5 FAM46C is induced in activated B lymphocytes and localizes mainly in the cytosol. a Splenocytes from FAM46C -FLAG +/+ knock-in mice and control animals were isolated and then cultured in presence of IL4 and LPS for 72 h. The level of FAM46C-FLAG was checked by western blot in non-activated (lanes 1–2) and activated (lanes 2–4) cells. GRP94 was used as activation marker, while DBC1 was used as a loading control. b Endogenous FAM46C localizes mainly in the cytosol. Splenocytes from WT and FAM46C -FLAG+/+ mice were isolated and fractionated. The whole-cell (T), cytoplasmic (CE), and nuclear (NE) extracts were analyzed by western blot. FAM46C-FLAG was detected using an anti-FLAG antibody. GAPDH and GRP94 were used as a cytosolic markers, while histone H4 and PSPC1 were used as nuclear markers. Arrow indicates the position of FAM46C-FLAG, while asterisks indicts nonspecific bands detected by antibodies, which were present in samples isolated from both WT and FAM46C-FLAG animals Full size image In order to study the potential role for FAM46C in B lymphocytes and more generally in hematopoiesis, we have generated FAM46C mutant animals, which harbor a 17 bp deletion and a 301 bp insertion using the CRISPR. This mutation causes a frameshift at position C88 and premature FAM46C protein termination, which takes place 26 amino acids after the breakpoint. Although, detailed analysis of FAM46C KO phenotypes are outside of the scope of this study, the mice did not display any major developmental phenotypes. However, we did detect several hematologic abnormalities (Fig. 6a–h ). Homozygous FAM46C KO mice ( FAM46C −/− ) had significantly lower hemoglobin level than age- and sex-matching FAM46C + /+ controls, suggesting that they suffer from anemia. The red blood cells count was also increased while MCV, MCH and MCHC were all significantly decreased. The microcytic and hypochromic erythrocytes imply that insufficiency of hemoglobin production is the most probable cause of the anemia. The MCV/RBC ratio (Mentzer index) is lower in FAM46C − / − (2.52) than in FAM46C +/+ (4.39), suggesting the anemia is a consequence of a block in globin synthesis rather than iron insufficiency. This hypothesis has to be further tested experimentally. These results are generally in agreement with the unpublished work from the Fleming laboratory described in the Meng Tian PhD thesis, but runs contrary to the Mouse Phenotypic Consortium, which has found FAM46C an essential gene. We suppose, that this discrepancy may be due to some linked lethal mutation generated by the consortium. Fig. 6 FAM46C KO 12-week-old mice display reduced blood hemoglobin levels and activated primary B lymphocytes proliferate faster. a – h Hematologic parameters of FAM46C KO and control animals: a Blood hemoglobin concentration (WT, n = 8; FAM46C KO, n = 6); b red blood cells count (RBC) (WT, n = 7; FAM46C KO, n = 7); c mean corpuscular volume (MCV) (WT, n = 10; FAM46C KO, n = 10); d mean corpuscular hemoglobin (MCH) (WT, n = 10; FAM46C KO, n = 10); e mean corpuscular hemoglobin concentration (MCHC) (WT, n = 10; FAM46C KO, n = 10); f blood platelets (WT, n = 9; FAM46C KO, n = 9); g Hematocrit (WT, n = 8; FAM46C KO, n = 8); h bone marrow (BM) plasmocytes (WT, n = 12; FAM46C KO, n = 12). P -values were calculated using two-way ANOVA tests (** P < 0.01, **** P < 0.0001). i Analysis of the proliferation rate of activated primary B cells. B lymphocytes isolated from FAM46C KO mice and matching WT controls were stained with CFSE and in vitro activated using IL4 and LPS. Cell divisions were monitored by levels of CFSE dilution. One representative experiment of 2 is presented. For each experiment splenic B lymphocytes from three individuals have been pulled, for both WT and mutant mice Full size image Importantly, analysis of in culture-activated primary splenic B lymphocytes revealed that FAM46C mutation leads to an increased proliferation rate, what indicates that FAM46C decreases the growth rate of B cells (Fig. 6i ). In conclusion, FAM46C acts as a growth suppressor not only for MM cells but also more generally in B-cell lineage cells. FAM46C polyadenylates multiple ER-targeted protein mRNAs In order to identify FAM46C substrates in MM cells, deep sequencing of total RNA from SKMM1 and H929 MM cell lines was performed after 3 days of FAM46C WT -GFP and FAM46C mut -GFP overexpression. RNA samples were prepared in triplicates or quadruplicates and depleted of rRNA, and strand-specific total RNA libraries were prepared. The samples were sequenced and mapped to an average depth of 15 million uniquely aligning reads. Differential expression analyses revealed significant differences in transcriptomes and responses to FAM46C expression among tested MM cell lines (Fig. 7a, b and Supplementary Data 1 ). When FAM46C was overexpressed, H929 cells had an increase in steady-state levels of many transcripts that encode proteins involved in the interferon response. This effect was not observed in the SKMM1 cell line. Nevertheless, there was a significant overlap (538 mRNAs) between upregulated transcripts among MM cell lines (Fig. 7c ). Notably, functional annotation clustering analysis of upregulated transcripts in SKMM1 and H929 MM cells expressing FAM46C WT (FDR < 1%), (using DAVID) revealed significant enrichment towards transcripts encoding proteins that pass through ER/Golgi and are transported into lysosomes or exported outside the cell (Fig. 7d and Supplementary Fig. 7a, b ). Fig. 7 Global analysis of FAM46C substrates in MM cells. a , b MAplots of total RNA sequencing results representing differential expression analysis of FAM46C WT -GFP and FAM46C mut -GFP-transduced MM cell lines. SKMM1 ( a ) and H929 ( b ) show transcriptome wide moderate deregulation of gene expression. Statistically significant values (FDR < 1%) are shown in red . The 396 transcripts constituting the common part for SKMM1 and H929 MM cell lines are marked with green circles . c Venn diagram demonstrating the overlap between upregulated transcripts in SKMM1 and H929 MM cell lines. d Functional GO terms annotation clustering of significantly upregulated transcripts in both MM cell lines. e , f Histogram representing the distribution of FAM46C-dependent polyadenylation rations monitored in fraction #5 ( e ) and #6 ( f ) in SKMM1 cell lines. Modeled normal distribution is fitted as a red line to emphasize the outlying population of FAM46C polyadenylated transcripts. g Venn diagram demonstrating the overlap between transcripts shifting to both long poly(A) fractions in FAM46 WT overexpressing cells mutually in SKMM1 and H929 MM cell lines. h 396 transcripts constituting the common part for SKMM1 and H929 MM cell lines were used in DAVID Functional Annotation Clustering Analysis. i The same set of transcripts was used to characterize the 3′-UTRs and total mRNA lengths showing a bias towards shorter species in either Full size image In order to take a closer look at changes after wild-type FAM46C expression, we fractionated mRNA based on poly(A) tail length from H929 and SKMM1 MM cells expressing FAM46C WT -GFP, FAM46C mut -GFP, and GFP for 72 h. RNA-seq libraries were prepared from two RNA fractions with the longest tails (fractions 5 and 6) and one fraction with the shortest poly(A) tail (fraction 1), followed by library preparation, sequencing, and initial analysis (analogous to the one described for RNA-seq). In order to identify FAM46C substrates, we aimed to determine differences in the enrichment of mRNA species in the highly polyadenylated fractions in cells transduced with wild-type FAM46C compared to cells transduced with the catalytically inactive mutant. To this end, we calculated “polyadenylation ratios” by dividing the levels of individual mRNA in long poly(A) fractions (5 and 6) relative to the short fraction 1 in FAM46C WT cells using relative levels observed in FAM46 C mut cells. Plotting the histograms of polyadenylation ratios revealed a significant set of transcripts with elongated poly(A) tails, which did not fit the normal distribution (Fig. 7e, f and Supplementary Fig. 7c, d ). This approach allowed us to identify 1744 mRNAs for SKMM1 and 659 mRNAs for H929 that shift towards longer poly(A) fractions in response to forced FAM46C WT expression; thus, they are presumably polyadenylated by this protein. The top-scoring transcripts were compared and as much as 60% of all H929 statistically significant hits were in common with SKMM1 hits, suggesting strong substrate specificity of FAM46C (Fig. 7g and Supplementary Data 2 ). Moreover, in the case of SKMM1 cell line the levels of basically all polyadenylated transcripts were increased confirming the role of FAM46C -mediated polyadenylation in enhancing mRNA stability. The correlation between the polyadenylation and mRNA levels was also visible for H929 MM cells. The effect, was, however, less pronounced, most probably due to the interferon response observed in H929—but not in SKMM1—which is known to have a strong influence on transcriptome hemostasis. Importantly, clustered GO-term analysis of transcripts polyadenylated by FAM46C using DAVID ( https://david.ncifcrf.gov/ ) revealed that, as in the case of standard RNA-seq analysis, many FAM46C substrates encode proteins that pass through ER/Golgi and are transported into lysosomes or exported outside the cell (Fig. 7h ) [21] , [22] . Moreover, despite filtering for highly-expressed transcripts in an analysis that usually creates a bias towards longer mRNAs, we found that short mRNAs with short 3′-UTRs are more prone to being substrates of FAM46C (Fig. 7i ). Sequence analysis of 3′-UTRs of FAM46C -polyadenylated mRNA revealed that, although not a single specific-sequence motif could be identified, there was a striking enrichment of highly statistically significant GpU- and CpU-rich motifs compared to 3′-UTRs of all expressed genes (Supplementary Fig. 7e ). These motifs or secondary structures may be recognized by FAM46C directly or indirectly through other recruiting factors. SSR4 (signal sequence receptor subunit delta), which is involved in the translocation of proteins across the endoplasmic reticulum membrane, was identified as a top hit FAM46C substrate in both MM cell lines. SSR4, as well as other ER-targeted proteins, such as CD320 , NAPSA , and FTL , were selected for further validation analysis based on the fact that ER stress is considered to be one of the most important processes in maintaining and targeting MM cells and augmentation of ER overload by proteasome inhibitors has emerged as an important therapeutic strategy for MM treatment. Northern blot analysis confirmed that SSR4 , CD320 , and FTL transcripts migrate much slower, as their poly(A) tails are extended in H929 and SKMM1 MM cells expressing FAM46C WT -GFP (Fig. 8a ); this effect was not observed when GFP only or FAM46 mut -GFP were expressed. Moreover, poly(A) tails were not extended in other cell lines derived from hematological malignancies, such as in Raji and HL60 transduced with FAM46C . Furthermore, SSR4 mRNA is polyadenylated at the 3′ end as revealed by analysis using RNase H cleavage assay with oligo(dT)25 followed by northern blot (Fig. 8b ); similar molecular phenotypes were determined for the translocon-associated protein SSR2 (Signal Sequence Receptor, Beta) (Supplementary Fig. 8a, b ). Fig. 8 FAM46C expression results in polyadenylation of selected mRNAs in MM cells. a Northern blot analysis of SSR4 , CD320 , and FTL transcripts from H929 (lanes 1–3), SKMM1 (lanes 4–6), Raji (lanes 7–9) and HL60 (lanes 10–12) cells transduced with GFP (lanes 1, 4, 7, 10), FAM46C WT -GFP (lanes 2, 5, 8, 11), and FAM46C mut -GFP (lanes 3, 6, 9, 12). Asterisks indicate cross-hybridization signals. b The SSR4 transcript is extensively polyadenylated by FAM46C in MM cells. High-resolution northern blot analysis of SSR4 transcripts from SKMM1 (lanes 1–6) and H929 (lanes 7–12) transduced with GFP (lanes 1, 2, 7, 8), FAM46C WT -GFP (lanes 3, 4, 9, 10), and FAM46C mut -GFP (lanes 5, 6, 11, 12) after RNase H treatment (lanes 1, 3, 5, 7, 9, 11) to remove the poly(A) tail in presence of oligo(dT) 25 . Control reactions were carried out in the presence of oligo(dT) without RNase H (lanes 2, 4, 6, 8, 10, 12). Kinetics of polyadenylation of SSR4 , NAPSA , FTL , and CD320 transcripts over the time course of FAM46C expression. c High- and low-resolution northern blot analysis of SSR4 , NAPSA , GAPDH , and RN7 transcripts from H929 (lanes 1–7) and SKMM1 cells (lanes 8–14) transduced with FAM46C WT -GFP up to 24 h. d High-resolution northern blot analysis of SSR4 and FTL transcripts from H929 (lanes 1–8) and SKMM1 cells (lanes 9–16) transduced with FAM46C WT -GFP (lanes 1–4, 9–12) and FAM46C mut -GFP (lanes 5–8, 13–16) up to 72 h. e Northern blot analysis of NAPSA and CD320 transcripts from H929 (lanes 1–4) and SKMM1 cells (lanes 5–8) transduced with FAM46C WT -GFP up to 72 h Full size image Additionally, poly(A) tail length dynamics of selected mRNAs during FAM46C expression were also evaluated in a time course. Cells were transduced with FAM46 WT -GFP and FAM46C mut -GFP, collected at indicated time points, and analyzed using northern blot. The first extended molecules were detected after 16 h of FAM46C WT -GFP expression in both cell lines (Fig. 8c–e ). In order to determine if the effect of SSR4 mRNA polyadenylation was specific to the FAM46C protein, we constructed lentiviral vectors allowing for expression of other RNA poly(A) polymerases, including GLD2-GFP, PAPOLA-GFP, and POLS-GFP, and transduced H929 and SKMM1 cells, and confirmed that this phenotype is caused by expression of FAM46C gene (Supplementary Fig. 8c ). It was concluded that FAM46C polyadenylates a broad spectrum of substrates in MM cell lines, inducing strong enrichment in those encoding ER-targeted proteins. FAM46C is a monomer and co-purifies with BCCIPβ and PABPC1 Cytoplasmic non-canonical poly(A) polymerases usually obtain specificity through associated RNA-binding proteins [23] , [24] . In order to identify the proteins interacting with FAM46C , co-immunoprecipitation (Co-IP) experiments were performed using SKMM1 and H929 MM cells expressing FAM46C WT -GFP. High-resolution mass spectrometry (MS) followed by label-free quantification (LFQ) revealed that BCCIPβ is the only protein enriched in both MM cell lines (Fig. 9a , Supplementary Data 3 ). Analyses performed in HEK293 cells also allowed for the identification of cytoplasmic poly(A)-binding protein PABPC1 as a potential FAM46C interactor (Fig. 9b , Supplementary Data 3 ). PABPC1 was an interesting target due to the poly(A) polymerase enzymatic activity of FAM46C . Interactions between FAM46C and BCCIPβ, PABPC1 were confirmed by Co-IPs followed by western blot analyses of HEK293, SKMM1, and H929 MM stable cell lines expressing FAM46C WT -GFP. Interaction of FAM46C with BCCIPβ was very stable under all experimental conditions tested; however, interaction with PABPC1 was identified only at physiological salt concentration (Fig. 9b ). Despite the fact that HEK293 cells express both FAM46A and FAM46B proteins, none of these co-purified with FAM46C, suggesting that they do not form heteromers. Fig. 9 FAM46C interacts with BCCIPβ and PABPC1 in human cells. a Visualizations of Co-IP-MS experiments using GFP-tagged FAM46C expressed in myeloma cells H929 (shown in blue ) and SKMM1 (shown in red ). Estimated quantities of identified proteins were calculated using the label-free quantification (LFQ) algorithm and are represented as dot–plot graphs. Protein abundance was calculated as LFQ intensity of the protein signal divided by its molecular weight and is shown on the x axis on a logarithmic scale. Specificity was defined as the ratio of protein LFQ intensity measured in the bait Co-IP to the background level (protein LFQ intensity in a sample) and is shown on the y axis on a logarithmic scale. b , c Western-blot detection of BCCIPβ and PABPC1 co-immunoprecipitated with: b FAM46C WT -GFP and FAM46C mut -GFP from stable HEK293 cell lines; c FAM46C WT -GFP from transduced SKMM1 and H929 MM cell lines. Purification was performed at low (lanes 1–3) and high (lanes 4–6) ionic strengths. GFP-tagged FAM46C was detected with α-GFP antibodies. Please note that the lack of the GFP signal in the GFP only control (lanes 1 and 4) is because the blot was cutoff to avoid very strong GFP signal, which could influence the readout Full size image PABPC1 and BCCIPβ proteins were selected for functional evaluation as potential FAM46C interactors. First, it was determined whether these proteins had any impact on mRNA after tethering to an RL reporter construct. Similarly to previous experiments, cells were transiently transfected with pRL-5BoxB, pNHA-BCCIPβ, and pNHA-PABPC1 plasmids and, after 24 h, RL mRNA and protein levels were analyzed. BCCIPβ did not affect mRNA; however, PABPC1 tethering led to increased RL mRNA and protein levels (Supplementary Fig. 9a–c ). Next, we examined FAM46C poly(A) polymerase activity in cells with reduced BCCIP and PABPC1 levels after siRNA treatment. HEK293 cells were treated with siRNA against BCCIP or PABPC1 mRNAs and, after 3 days, reseeded and co-transfected with pRL-5BoxB, pNHA-FAM46C, and pNHA-FAM46C mut . BCCIPβ and PABPC1 protein levels after siRNA treatment were determined by western blot analysis (Supplementary Fig. 9d ). After 24 h, steady state levels of reporter mRNA and protein were analyzed (Supplementary Fig. 9e ). In all cases, FAM46C tethering led to increases in steady state RL mRNA and protein levels (Supplementary Fig. 9e ). In conclusion, FAM46C does not form stable macromolecular assemblies and interacting proteins have no direct effect on its poly(A) polymerase activity. Thus, the mechanism through which FAM46C gains specificity towards particular mRNAs remains unknown. Template-independent elongation of the 3′-end of mRNA by nucleotidyltransferases, known as poly(A) polymerases, plays a crucial role in RNA processing that affects mRNA stability and translational efficiency. Here we provide strong in vitro and in culture evidence demonstrating that the FAM46C gene encodes a novel poly(A) polymerase that acts as an B-cell lineage growth suppressor. Reintroduction of FAM46C into MM cell lines with dysfunctional endogenous gene leads to cell death while its silencing in cells expressing WT proteins enhances proliferation rate. Furthermore, activated primary B lymphocytes isolated from FAM46C KO animals divide faster than the wild type, suggesting that FAM46C acts more generally in the B lymphocyte lineage. Hematologic phenotypes of FAM46C KO animals, in which red blood cell and platelet counts are increased further suggests that this enzyme controls proliferation of other blood cells or common progenitor. To summarize, we are strongly confident that MM cells must benefit from mutations in FAM46C, however we cannot exclude that FAM46C suppresses the growth of other cell types than ones derived from the B-cell linage. Recent studies from the Xin Lab suggest that FAM46C can also be involved in regulation of proliferation of hepatocellular carcinoma cells [25] , [26] . Our data based on SKMM1 and H929 cell lines strongly indicate that FAM46C has a relatively broad spectrum of substrates with significant enrichment towards ER/Golgi-targeted proteins, which may explain the toxicity to MM cells since ER and Golgi apparatus homeostasis is essential for survival. Although we did not determine the specificity of the FAM46C protein for particular substrates, we found that the toxicity of FAM46C to MM cells is unique, since overexpression of other poly(A) polymerases, such as GLD2 and canonical PAP, was not harmful to MM cells. Similarly to the overexpression of the wild-type form of FAM46C in HL60, there was no significant effect on the survival of Raji and 293 T cell lines. These results suggest that the toxicity of FAM46C to MM cell lines is related to the expression of ER/Golgi-targeted proteins, which may result in ER overload and induction of an unfolded protein stress response in these cells [27] , [28] . However, how exactly the numerous genetic differences between cancer cell lines makes them sensitive to FAM46C expression remains to be established. Importantly, this work provides the first experimental evidence directly linking RNA 3′ end polyadenylation process with cell proliferation, notably in the B-cell lineage implying the possible role of FAM46C mutations as driver mutations in MM. Interestingly, a well-established regulator of polyadenylation in gametogenesis, cytoplasmic polyadenylation element binding (CPEB), is also implicated in senescence and was suggested to be a tumor suppressor [29] , [30] , [31] . However, the enzyme responsible for CPEB-dependent polyadenylation in somatic cells remains unknown, as knock-out of the poly(A) polymerase GLD2, which cooperates with CPEB in Xenopus oocytes [32] , [33] , has no visible phenotype in mice [34] . PABPC1 and BCCIP proteins are novel FAM46C interactors that had not been reported in high throughput screens. The cytoplasmic-nuclear shuttling protein PABPC1 is a FAM46C interactor and is directly related to its physiological function, since it binds to nascent poly(A) tracts, affecting initiation of protein translation and both RNA processing and stability; however, the additional factors determining FAM46C substrate specificity require further investigation. Furthermore, FAM46C displays very weak distributive activity in vitro, while it seems to be more active in vivo, thus additional factors responsible for its optimal activity probably remain to be identified. Our identification of FAM46 proteins as active poly(A) polymerases suggests that the human genome encodes at least 11 putative ncPAPs and PUPs (4 FAM46 family members and 7 other previously annotated genes; Table 1 ). FAM46C, as well as all other members in this family, may positively regulate gene expression in various human tissues and organs, since they are differentially expressed during development and several tissues express multiple FAM46 proteins at the same time [35] . Further research is necessary in order to determine the physiological roles of this novel family of poly(A) polymerases. Data obtained thus far strongly suggest that gene expression regulation by cytoplasmic polyadenylation may play a role in various other cellular processes. Our initial analysis of FAM46C KO animals suggests several hematologic abnormalities, like anemia, what is in agreement with previously reported data. However, how exactly FAM46C affects erythropoiesis remains to be established. Table 1 List of human non-canonical PAPs and PUPs Full size table Recent studies have shown that loss-of-function mutation within FAM46A is associated with bone abnormalities in mice and in autosomal recessive retinitis pigmentosa in humans; however, its molecular function remains unexplained [6] , [12] , [36] , [37] . FAM46A is expressed in the ameloblast nuclei of tooth germs and may be important for the formation of enamel in teeth [38] . The FAM46A sequence polymorphisms SNP (rs11040) and VNTR, within its coding sequence in exon 2 (15bp VNTR repeats may vary from two to seven repeats), were also associated with a susceptibility to tuberculosis [39] . FAM46A expression has been reported to increase over two-fold in macrophages after stimulation by heat-attenuated Mycobacterium tuberculosis (H37Rv). The VNTR polymorphism in the FAM46A gene has also been associated with susceptibility to large-joint osteoarthritis (hip and knee) and non-small cell lung cancer [40] , [41] . FAM46D expression is strongly upregulated in transgenic mice (MALTT) that exhibit autism spectrum disorder-like behaviors (ASD) [42] . Since FAM46 proteins are active poly(A) polymerases, these data strongly suggest that additional phenotypes may be related to the regulation of posttransciptional gene expression. In conclusion, this study identified that the human FAM46C gene encodes a novel poly(A) polymerase and showed FAM46C potential to regulate gene expression posttranscriptionaly resulting in an significant impact on several cell types in the hematopoetic lineages in mice. Thus, demonstrating importance of RNA poly(A) tail homeostasis for cancer cell survival which could be further pursued as a potential therapeutic target for MM treatment. Cell lines MM cell line SKMM1 was kindly provided by W. Michael Kuehl, M.D., Genetics Branch Head, Molecular Pathogenesis of Myeloma Section National Cancer Institute), H929 (ATCC; CRL-9068), MM1.S (ATCC; CRL-2974), MM1.R (ATCC; CRL-2975), RPMI8226 (ATCC; CCL-155), and Raji Burkitt’s lymphoma (ATCC; 85011429) were cultured in RPMI 1640 ATCC’s modified (Invitrogen) supplemented with 10% FBS (Invitrogen) and penicillin/streptomycin (Sigma; P4083). HL60 cells were cultured in IMDM (Invitrogen) with 20% fetal bovine serum (FBS) and penicillin/streptomycin. HEK293T (ATCC; CRL-3216), Flp-In-293 Cell Line (Invitrogen; R78007), HeLa (ATCC; CCL-2), and U2OS (ATCC; HTB-9) were cultured in Dulbecco’s modified Eagle’s medium (DMEM; Invitrogen) supplemented with 10% FBS (Gibco) and penicillin/streptomycin at 37 °C in 5% CO 2 . All cell lines were tested for mycoplasma contaminations upon arrival and routinely during their culture. Induction of stable cell lines was obtained by addition of tetracycline (Gibco) to a final concentration of 100 ng/ml. siRNAs and plasmid transfections were performed with Lipofectamine 2000 and Opti-MEM media (Invitrogen) according to the manufacturer’s instructions. For transcription inhibition, actinomycin D (Sigma; A9415) was added to a final concentration of 5 µg/ml at the times indicated. MM cell line genotyping The exon 2 of FAM46C gene was amplified using hFAM46C_ex2_1F and hFAM46C_ex2_1R primers, which were designed with Oligo software (MBI, USA) and Primer-Blast [43] . Purified PCR products were sequenced and then thoroughly analyzed with Mutation Surveyor 4.0 software (SoftGenetics) against the presence of mutations and other differences compared to GenBank reference sequences NC_000013 and NC_000001.11. The Mutation Surveyor allowed for detection of minor alleles down to 5%, basing analysis of both strands. Sequencing results are summarized in Supplementary Table 1 . General molecular biology techniques General molecular biology techniques were conducted as described in Molecular Cloning [44] . Low-molecular weight RNA samples were separated on 4–6% acrylamide gels containing 7M urea in 0.5× TBE buffer and transferred to a Hybond N+ membrane by electrotransfer in 0.5× TBE buffer. High-molecular weight RNA samples were separated on 1.2% agarose gels containing formaldehyde in 1× NBC buffer and transferred to membranes by capillary elution using 8× SSC buffer. After transfer membranes, blots were stained with 0.03% methylene blue in 0.3 M NaAc pH 5.3 for 10’ at room temperature, scanned and then destined with water. RNA was immobilized on membranes by 254 nm UV light using a UVP CL-1000 crosslinker. Radioactive probes were prepared with a DECAprime II DNA Labeling Kit (Invitrogen). Northern blots were carried out in PerfectHyb Plus Hybridization Buffer (Sigma), scanned with Fuji Typhoon FLA 7000 (GE Healthcare Life Sciences) and analyzed with Multi Gauge software Ver. 2.0 (FUJI FILM). All western blotting experiments were performed in accordance with the technical recommendations of the antibodies’ suppliers. 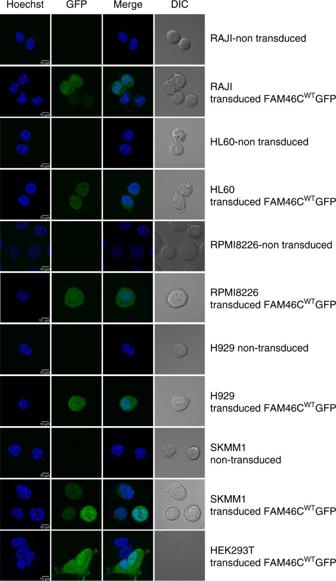Fig. 2 FAM46C shows both nuclear and cytoplasmic localization. HEK293T, RPMI826 (MM), H929 (MM), SKMM1 (MM), HL60 (promyelocytic leukemia) and Raji (B-cell lymphoma) cell lines were transduced with constructs encoding theFAM46CWT–GFP fusion gene. Non-transduced cells were used as a control. Fluorescence images for GFP and Hoechst nucleic acid stain, as well as merged images, are shown.Scales bars(10 µm) are shown for each set of images All antibodies used in this study are listed in Supplementary Table 2 . Unprocessed scans of selected major blots and gels are shown in the Supplementary Fig. 10 . Cloning and construct preparation The primers used for cloning are listed in the Supplementary Data 4 . All plasmid-encoding constructs for tethering assays and miRNA were cloned using classical restriction enzyme digestion and ligation approaches; all other constructs were prepared with SLIC [45] , [46] . The pClneo-NHA vector and pRL-5BoxB (Renilla luciferase containing five BoxB structures) were kindly provided by Prof. Witold Filipowicz (FMI). pNHA-GENE constructs were prepared using classical restriction ligation methods. All pcDNA-GENE-TEV-eGFP constructs were prepared by PCR amplification from human cDNA using the appropriate primers listed in Supplementary Data 4 . PCR products were subsequently cloned into a modified version of the pcDNA™5/FRT/TO vector (Invitrogen) using the SLIC method. Plasmid pcDNAFAM46CmutGFP was obtained by site-directed mutagenesis using the pcDNAFAM46CmutF and pcDNAFAM46CmutR primers with the pcDNAFAM46C WT GFP plasmid served as a template; final constructs were verified by sequencing. The HA-tag was inserted into pKK-NoTag made in PCR reaction with primers N_Met-HA_for and N_Met-HA_rev using Acc65I and BamHI cut pKK-NoTag and then assembled with SLIC approach giving pKK-HA. pKK-NoTag is a modified version of pcDNA5FRTTO (All additional information will be described in forthcoming publication). pKK-HA-FAM46C construct was cloned using classical restriction ligation protocol into pKK-HA BshTI and NheI restriction sites. To obtain pCI-NHAFAM46DWT and pCI-NHAFAM46Dmut PCR product with primers NHFAM46DF and NHFAM46DR and pKK-FAM46DWT or pKK-FAM46Dmut plasmids, respectively and cloned into EcoRI and NotI sites in pCI-NHA vector. All SFFV (pLVX) lentiviral constructs were prepared in modified HIVSFFVRFP plasmids, which was kindly provided by Dr Verhoeyen Els (ENS de Lyon). All GENE-TEV-eGFP inserts were obtained from a PCR reaction with the appropriate plasmid pcDNA-GENE-TEV-eGFP and universal SFFV_F and SFFV_R primers. PCR products were cloned into the plasmid HIVSFFVRFP and digested by BamHI and XhoI using the SLIC protocol. To make HIVSFFV-NHA-FAM46C construct, PCR product with primers 15_129_F and 15_129_R and pCI-NHAFAM46C plasmid as template was cloned into HIVSFFV vector using SLIC approach. To obtain HIVSFFV FLAG-FAM46C construct, PCR product with primers 15_125F1 and HivN_R using pCDNA FAM46CGFP plasmid as template, then reamplified with HivNFlgF and HivN_R and finally was cloned into HIVSFFV vector using SLIC. To make HIVSFFV-RL and HIVSFFV-FL constructs, PCR products obtained with primers 15_131nF/15_131R1 and 15_133_F/15_133_R using pRL-TK (Promega) and pGL3-Control (Promega) templates were cloned into HIVSFFV vector using SLIC approach. To obtain HIVSFFV-RL5Box construct, two PCR product with primers 15_131nF/15_131R1 and 15_131F2/15_131_R using pRL5Box (from Prof. Filipowicz) plasmid as template were cloned in one reaction into HIVSFFV vector using SLIC approach. The HIVSFFV FAM46C-FLAG constructs, was obtained by cloning of PCR product with primers HIV_for and 15_127R1 using pcDNA FAM46CGFP plasmid as template, then reamlified with HIV_for and HivCflgR and finally was cloned into HIVSFFV vector using SLIC approach. To make HIVSFFV GFP-FAM46C construct, GFP sequence was amplified with primers HivNgfpF and 15_127R1, FAM46C was amplified with primers 9_114_F and HivN_R using pCDNA FAM46CGFP plasmid as template for both reactions and finally was cloned into HIVSFFV vector in the same reaction using SLIC approach. All HIVSFFV construct were sequenced from HIV_f, HIV_r. Lentiviral packaging (pMD2.G) and envelope (pPAX2) plasmids were kindly provided by Prof. Didier Trono (École Polytechnique Fédérale de Lausanne, Switzerland). The FAM46CWT, FAM46DWT, and FAM46Cmut constructs for recombinant protein production in Escherichia coli BL21-CodonPlus-RIL strain (Stratagene) were prepared by PCR amplification from previous pcDNA constructs using appropriate primers. The PCR products were subsequently cloned into a modified pET28 vector using the SLIC method, resulting in N-terminal HIStag-SUMOtag fusion. Tethering assays Tethering assays were performed as previously described [19] . In brief, a day before transfection, 0.75 ml of HEK293 cells were seeded on 6-well plates to achieve about 70–80% confluence on the day of transfection. Next, cells were co-transfected with 100 ng of constructs expressing reporter Renilla luciferase (RL-5BoxB or RL), 100 ng of control firefly luciferase (FL, pGL3 plasmid) and 2 µg of plasmid encoding tethered NHA-protein using 5 µl of Lipofectamine 2000 and OPTI-MEM media (Invitrogen) according to manufacturer’s instructions. All transfections were repeated at least three times. Twenty-four hours after transfection, cells were collected, lysed and protein levels were analyzed by western blot. If transfected cells were used solely for the analyses of RNA they were co-transfected only with 0.1 µg pRL-5Box plasmid carrying Renilla luciferase (RL) and 2 µg of plasmid encoding tethered NHA-protein cells and then were collected 24 h after transfection. This approach was used to avoid trans effects between promoters on co-transfected plasmids which may affect RL reporter gene expression [47] . For special purposes, such as higher yield of RNA, cell cultures and transfections were scaled-up. Tethering assay in MM cells SKMM1 and H929 cells were co-transduced with lentiviral particles carrying FL and RL or RL5Box and FL at MOI 1. Expression of reporter genes in obtained stable cell lines was verified by western blot then cells were transduced with lentiviruses allowing expression of wild-type and mutated NHA-tagged FAM46C protein at MOI 5. Twenty-four hours after transduction, cells were collected and protein levels was determined by western blot. Gene silencing by siRNA and shRNAs siRNA-mediated knock-downs were performed using validated Stealth RNAi and Lipofectamine RNAiMAX (both Invitrogen) as previously described [48] . 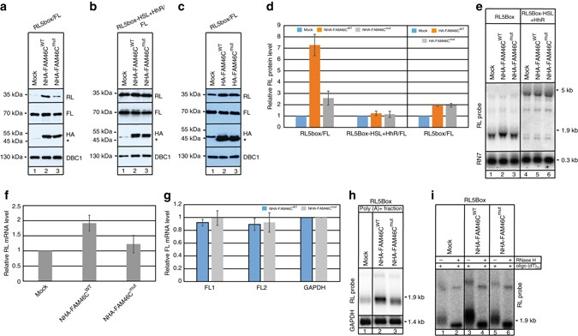Fig. 3 FAM46C tethering leads to polyadenylation and enhanced expression of aRenillaluciferase (RL) reporter. Analysis at the protein level (a–d):aFAM46C tethering increases RL reporter protein levels. HEK293 cells were co-transfected with a construct expressing RL, containing five boxB sites in its 3′-UTR, Firefly luciferase (FL) control reporter and FAM46CWTharboring the N-terminal λN boxB-binding domain and HA-tag. Western blot detection of RL in mock-transfected cells (lane 1) and after NHA-FAM46CWT(lane 2) or NHA-FAM46Cmut(lane 3) tethering. Expression of NHA-tagged FAM46C proteins were confirmed using an α-HA antibody. DBC1 served as a loading control.Asterisksindicate cross-hybridization signals.bExpression of RL5boxHSL + HhR reporter with a cyclic phosphate at the 3′ end generated by a hammerhead ribozyme was not enhanced upon FAM46C tethering. The experiment was performed as ina.cExpression of the FAM46C without λN domains did not enhance expression of the reporter. The experiment was performed as ina.dQuantifications of RL protein normalized by the internal FL reporter related to experiments froma–c. RNA analysis (e–i):enorthern blot detection ofRL mRNAusing total RNA from HEK293 cells after tethering of NHA-FAM46CWTor NHA-FAM46Cmutto RL5box (lanes 1–3) or RL5boxHSL + HhR with a cyclic phosphate at the 3′ end (lanes 4–6).fQuantifications of RL mRNA.gRT-qPCR analysis of the FL control reporter.hNorthern blot detection ofRenillaluciferase using poly(A) + fraction from HEK293 cells after tethering of NHA-FAM46CWTor NHA-FAM46Cmut(i) Poly(A) tails added to reporter mRNA can be removed by RNase H treatment in the presence of oligo(dT)25. High-resolution northern blot analysis of RL mRNA from control HEK293 cells (lanes 1–2), after tethering of NHA-FAM46CWT(lanes 3–4) or NHA-FAM46Cmut(lanes 5–6). The data ind,f,gare shown as a mean value ± SD (n= 3) For silencing of BCCIP and PABPC1, three different siRNAs were tested; they are listed in Supplementary Table 3 . For further analyses, cells were collected or re-plated 72 h after transfection. 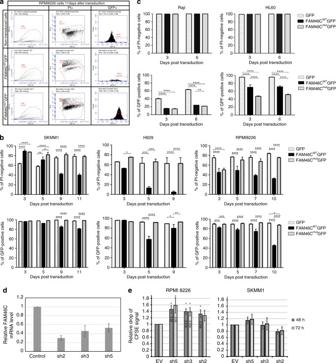Fig. 4 FAM46C control survival and proliferation of multiple myeloma cells.a–cExpression ofFAM46CWTinduces death in multiple myeloma cells.aAn example gating strategy for defining transduction efficiency and cell viability. Forward scatter (FSC) and side scatter (SSC) gate were used to separate debris from intact cells. Viability of RPMI8226 cells overexpressing either FAM46CWT-GFP or FAM46Cmut-GFP was analyzed using propidium iodide (PI) staining on the 11th day post-transduction. GFP expression (GFP+) was evaluated in parallel in PI-negative cells.b,cSummary of flow cytometry analyses presented as bar graphs showing GFP expression level and reduced viability of multiple myeloma cell lines (SKMM1, H929, and RPMI8226 inband Raji and HL60 incthroughout the time course of GFP, FAM46CWT-GFP, and FAM46Cmut-GFP expression. The data are presented as percentage of cells ± SD (n= 3).Pvalues were calculated using two-way ANOVA tests (*P< 0.05, **P< 0.01, ***P< 0.001, ****P< 0.0001).d,eshRNA-mediated silencing ofFAM46Cenhances proliferation rate of RPMI8226 MM cell line expressing wild-type protein but not SKMM1 harboring FAM46C mutation. Cells were transduced with lentiviral vectors expressing shRNA and empty vector as control. Stable transduced cell lines were stained with CFSE. Cell division was monitored by flow cytometry after 48 and 72 h by levels of CFSE dilution.dReverse transcription qPCR analysis of the FAM46C silencing efficiency.Barsrepresent mean values ± SD (n= 3).eThe rate of proliferation of shRNA treated cells normalized to the control transduction.Barsrepresent mean values ± SD.P-values were calculated using Student’st-test (*P< 0.05), (n= 3) The shRNA against human FAM46C were purchased from Sigma Aldrich and are listed in Supplementary Table 4 . Lentiviral particles were obtained and triter as described below in “Transduction of target cells” section. Cells were transduced at MOI 1 and the third day after transduction were subjected to selection with puromycin (Invitrogen) at 0.5 µg/ml (for H929) and 1 µg/ml (for SKMM1 and RPMI8226) for 7 days to obtain stable cell lines. The level of remaining transcript was determinate by RT-qPCR. B cells and MM cells proliferation assay Naive B cells have been isolated from 3 polled spleens of sex-matched 12-weeks-old littermate mice using CD43 microbead (Miltenyi Biotec) negative selection and were cultured in RPMI 1640 containing 15% FBS. B cells were activated by the addition of 20 µg/ml LPS (Sigma) and IL-4 (R&D Systems) at 20 ng/ml to the culture media. Both primary murine B-cells and human MM cell lines have been stained with 5 μM CFSE according to manufacturer’s instructions and cultured for 72 h or 48 and 72 h, respectively. To calculate the rate of CFSE fluorescent signal dilution autofluorescence, defined as the signal from unstained samples, have been subtracted from the fluorescence of the stained cells and initial (0 h) values have been divided by ones measured at 48 and 72 h. The results were presented as relative to the control transfected with an empty vector. FAM46C localization The 293T, RAJI, HL60, H929, SKMM1, RPMI8226 cells were transduced with lentiviruses caring FAM46C WT at MOI 1. Forty-eight hours after transduction cells were stained with Hoechst 33342 and subsequently processed. Non-transduced cells were used as auto fluorescence controls A day prior to transfection, cells were seeded to Nunc™ Lab-Tek™ II Chamber Slide™ Systems in order to reach 50% of confluence on the day of transfection. DNA was stained by adding the dye Hoechst 33342 (Invitrogen) to the medium to a final concentration of 2 mg/ml. After 20 min of incubation at 37 °C, the medium was exchanged and cells were prepared for observation. For the intravital observation of the cells, a confocal system (Fluoview FV1000) equipped with a spectral detector (Olympus) and a 60×/1.2 water immersion objective was used. Images were processed using ImageJ software. RNA isolation and poly(A) fractionation RNA isolation was performed with TRIzol reagent (Invitrogen, 15596) according to the manufacturer’s instructions. Poly(A) fractionation was performed as previously described with the following modifications [49] . In brief, 80 µg of total RNA was mixed with 400 µl GTC buffer (4 M guanidine thiocyanate, 25 mM sodium citrate, pH 7.1, 2% β-mercaptoethanol) and 750 pmol of 5′-biotinylated TEG-oligo(dT) 25 (Future Synthesis). 850 µl of “dilution buffer” (6 × SSC, 10 mM Tris-HCl, pH 7.4, 1 mM EDTA, 0.25% SDS, 1% β-mercaptoethanol) was added, the mixture was incubated at 70 °C for 5 min, and then it was centrifuged at 12,000 rpm for 10 min at RT. The resulting supernatant was mixed with 100 µl of M280 beads (Invitrogen; 60210) washed 3 times with 0.5 × SSC buffer. After binding, samples were washed 3 times with 0.5 × SSC buffer for 10 min. RNA fractions were eluted with decreasing concentrations of SSC buffer (from 0.2 × SSC to 0.025 × SSC) and the final elution was performed with water. RNA was precipitated and subjected to further analysis. RNAse H assay 20 µg of total RNA was mixed with 100 ng of oligo(dT) 25 (Invitrogen), heated for 1 min at 95 °C, and transferred to ice. Then, 10 µl of 5× RH buffer (100 mM, 0.5 M KCl, 50 mM MgCl 2 , 50 mM DTT, and 25% sucrose) was added to 5 U of RNaseH (NEB). Reactions were carried out for 45 min at 37 °C and RNA was recovered by extraction with phenol/chloroform, precipitated, and analyzed using northern blots. RNA-seq libraries 1 µg of total RNA was treated with Turbo-DNase (Life Technologies) according to the manufacturer’s instructions. Then, rRNA was removed from samples using a Ribo-Zero Kit (Epicentre), according to the manufacturer’s protocol, and samples were spiked-in with external RNA (ERCC RNA Spike-In Mix; Life Technologies). For libraries prepared from poly(A)+ fractions, the ribo-depletion step was omitted. Finally, RNA libraries were prepared using a TruSeq RNA Sample Preparation Kit (Illumina) or a KAPA Stranded RNA-Seq Library Preparation Kit (Kapa Biosystems) according to the manufacturer’s instructions. Quality of libraries was determined by chip electrophoresis performed using the Agilent 2100 Bioanalyzer (Agilent Technologies, Inc.). Transduction of target cells For lentivirus production, 2.6 × 10 6 HEK-293T cells were seeded into 10 cm dishes 24 h prior to transfection in 10 ml of DMEM supplemented with 10% FBS (Invitrogen) and penicillin/streptomycin solution (Sigma). The lentiviruses encoding the gene of interest (GOI) were introduced to the packaging cells by calcium phosphate co-transfection with 8.6 µg of a GOI-containing vector HIV-SFFV and components of 2nd generation of packaging vectors, namely, 8.6 µg of psPAX2 packaging vector and 5.5 µg of pMD2.G envelope vector. The plasmids were resuspended in 450 µl of 300 mM CaCl 2 and added dropwise to 450 μl of 2 × concentrated HEPES-buffered saline (280 mM NaCl, 20 mM HEPES, 1.5 mM Na 2 HPO 4 , 10 mM KCl and 12 mM D-glucose pH 7.2) by vortexing. The precipitate was immediately added to the cell culture medium with gentle swirling. The medium was replaced with 6 ml of fresh DMEM 16 h post transduction. Virus-containing supernatants were collected 24 h later, centrifuged for 3 min at 300 × g , and filtered through 0.45 μm low-protein-binding filters (Millipore) Then, the supernatants were concentrated 10 × by centrifugation (3000 × g , 16 h, 4 °C). The titer of viral particles was estimated using a Lenti-X p24 Rapid Titer Kit (Clontech) according to the manufacturer’s protocol. Multiplication of infection (MOI) was calculated by dividing the vector titer for the number of cells transduced. Efficiency of transduction was determined by flow cytometry for GFP-expressing cells using an Accuri C6 benchtop cytometer (BD Biosciences). Additional staining with 2.5 µg/ml propidium iodide (Sigma-Aldrich) in PBS was performed to distinguish dead cells. If needed, to select GOI-expressing cells, sorting for GFP-positive cells using the Aria III cell sorter (BD Biosciences) was performed. RNA-seq data analysis Ribo-depleted total RNA isolated from mutant and wild type H929 cell line quadruplicates were used to prepare strand-specific libraries (dUTP RNA); Ribo-depleted total RNA isolated from mutant and wild type SKMM1 cell line triplicates were also used to prepare non-strand-specific TRUseq RNA libraries. These libraries were subsequently sequenced using an Illumina HiSeq sequencing platform to the average number of 18.5 million reads per sample in 100-nt pair-end mode. Poly(A) tail length fractionation libraries were sequenced to an average depth of in 75-nt pair-end fashion. Reads were mapped to the reference human genome (hg38) using STAR short-read aligner with default settings (version STAR_2.4.0) yielding an average of 80.2% uniquely mapped reads [50] . The quality control, read processing and filtering, visualization of the results, and counting of reads for the Genecode v22 comprehensive annotation was performed using custom scripts utilizing elements of the RSeQC, BEDtools and SAMtools packages [51] , [52] . Differential expression analyses were performed using the DESeq2 Bioconductor R package [53] . For the poly(A) fractionation data, a “polyadenylation ratio” was calculated by dividing the levels of individual mRNA in long poly(A) fractions (#5 and #6) relative to the short fraction (#1) in WT FAM46C cells by equivalent relative levels observed in FAM46C mut -GFP cells. Functional clustering of GO terms analysis was performed using DAVID [22] . The search for common sequence motif was performed using HOMER [54] and further analyzed by STAMP [55] . Multiple alignment Multiple alignments analyses were performed using PRofile ALIgNEment (PRALINE) ( http://ibivu.cs.vu.nl/programs/pralinewww/ ) [56] , [57] . Mass spectrometry analysis MS analysis were performed essentially as described [58] . Briefly, precipitated proteins were dissolved in 100 μl of 100 mM ammonium bicarbonate buffer, reduced in 100 mM DTT for 30 min at 57 °C, alkylated in 55 mM iodoacetamide for 40 min at RT in the dark, and digested overnight with 10 ng/ml trypsin (Promega) at 37 °C. Finally, trifluoroacetic acid was added at a final concentration of 0.1%. MS analysis was performed by LC-MS in the Laboratory of Mass Spectrometry (IBB PAS, Warsaw) using a nanoAcquity UPLC system (Waters) coupled to an LTQ-Orbitrap Velos mass spectrometer (Thermo Scientific). Peptides were separated by a 180-min linear gradient of 95% solution A (0.1% formic acid in water) to 35% solution B (acetonitrile and 0.1% formic acid). The measurement of each sample was preceded by three washing runs to avoid cross-contamination; the final MS washing run was searched for the presence of cross-contamination between samples. If the protein of interest was identified in the washing run and in the next measured sample at the same or smaller intensity, then the sample was regard as contaminated and these samples were excluded from final graphs. The mass spectrometer was operated in the data-dependent MS-MS2 mode and data were acquired in the m / z range of 300–2000. Data were analyzed with the Max-Quant (Version 1.5.3.12) platform. The reference human proteome database from UniProt was used. We also searched our data for protein isoforms (for example BCCIP alfa/beta) to determine which were present. Label-Free-Quantification (LFQ) intensity values were calculated using the MaxLFQ algorithm to estimate quantities of identified proteins and identified proteins were analyzed as follows. Protein abundance was defined as the LFQ value calculated by MaxQuant software for a protein (sum of intensities of identified peptides of a given protein) divided by its molecular weight. Specificity was defined as the ratio of the protein LFQ intensity measured in the bait purification to background level (i.e., protein LFQ intensity in the negative control purification with the background level was arbitrarily set to 1 for proteins not detected in the negative control). High values of both protein abundance and specificity indicated proteins that were enriched in the purification and thus suggested interactions. Common protein contaminations were removed from graphs. All MS analyses were performed at the Mass Spectrometry Laboratory, IBB PAS. Co-Immunopreciptation Cell collected from two 145 mm plates at a confluency of 80–90% were fleshly frozen, thawed on ice, and incubated for 30 min at 4 °C with gentle rotation in 3 ml LB buffer (20mM Tris, 150 mM NaCl, 0.5% Triton-X100, 1 mM DTT, 1 mM PMSF, 0.02 µM pepstatin A, 0.02 µg/ml chymostatin, 0.006 µM leupeptin, and 20 µM benzamidine hydrochloride supplemented with proteases and phosphatase inhibitors; Invitrogen). Next, lysates were sonicated for 30 min in Bioruptor Plus (Diagenode) (30s pulses with 30s intervals), after which they were cleared by centrifugation at 13,000 rpm and 4 °C for 15 min. Immunoprecipitations were performed using house-in made affinity slurry CNBr-activated SepFast MAG 4HF [Biotoolomics] coupled with house-in purified anti-GFP antibodies). After 2h of incubation, beads were washed six times with LB buffer and finaly washed with TEV buffer (10 mM Tris-HCl pH 7.4, 75 mM NaCl, and 1 mM DTT). Cleavage with TEV protease was conducted for 2 h at RT. Then, proteins were precipitated with PRM reagents (0.05 mM pyrogallol red, 0.16 mM sodium molybdate, 1 mM sodium oxalate, 50 mM succinic acid, and pH 2.5 (Sigma-Aldrich)) and then analyzed by MS. Polyadenylation assay 150 ng of purified recombinant protein was mixed with 32 P-labeled RNA substrate (A) 15 in the presence of 1 mM ATP (NEB), 2 U/µl RNasine (Fermentas), 0.5 mM Mg 2+ , or Mn 2+ (or both) in PAP buffer (25 mM Tris-HCl pH 7.0, 50 mM KCl, 0.02 mM EDTA, 0.2 mM DTT, 100 µg/ml BSA [Invitrogen], and 10% glycerol). Reactions were carried out at 37 °C and stopped at indicated time points by addition of equal volume of RNA loading dye (98% deionized formamide, 25 mM EDTA pH 8.0, 0.025% (w/v) xylene cyanol, and 0.025% (w/v) bromophenol blue). Reaction products were separated in 8 M urea/15% PAGE in 0.5× TBE. RNA-protein UV-crosslinking and immunoprecipitation FAM46C WT GFP crosslinking to RNA followed by immunoprecipitation was performed as described [59] . Briefly, five 145 mm plates of stable HEK293 Flp-In TREx cell line expressing FAM46C WT GFP at 90% confluency were irradiated with 254 nm UV light (2500 µj/cm 2 ; UVP Crosslinker). Protein cross-linked to RNA were then immunoprecipitated with anti-GFP resin, followed by RNA labeling with 32 P, SDS-PAGE complexes separation, transferred to the nitrocellulose membrane, staining with Ponceau S, and autoradiographed. Mice generation Basing on UCSC Mice GRCm38/mm10 Assembly, sgRNA (chimeric single-guide RNA) were designed as close as possible to the catalytic site of FAM46C gene to generate knock-out and to the STOP codon to generate FLAG-tag knock-in mice. According to the MIT CRISPR online design tool (crispr.mit.edu) our guides, located chr3:100473168-100473187 and chr3:100472250-100472273, reached score of 82 and 57 points, respectively, with very low risk of off-targets (for guide RNA sequences see Supplementary Data 4 ). For sgRNA T7 RNA Polymerase based synthesis we used mFam46C_mut_sgRNA_f primer for FAM46C knock-out line or mFam46C_FLAG_sgRNA_f primer for FAM46C-FLAG knock-in line and Universal_sgRNA_rev primers (underlined is T7 RNA polymerase promoter). Cas9 mRNA synthesis Streptococcus pyogenes Cas9 CDS was amplified from PX458 (pSpCas9(BB)-2A-GFP, Addgene Plasmid #48138) using T7_SpCas9_for and SpCas9_rev primers and subsequently transcribed with T7 RNA polymerase. Collection of zygotes Ethical approval for the procedures on animals was obtained from I Local Ethical Commission for Experiments on Animals in Warsaw (decisions no. 527/2013 and 176/2016). Embryos used in all experiments were isolated from F1(C57BL/6×CBA) mouse females, which were induced to superovulate by injection of 10 IU of PMSG (Pregnant Mare Serum Gonadotropin; Folligon, Intervet, Netherlands) and 10 IU of hCG (Human Chorionic Gonadotropin; Chorulon, Intervet, Netherlands) 48–52 h later. Females were mated with males of the same strain immediately after hCG injection. Zygotes were collected from mated females 21–22 h post hCG injection. They were released from the oviducts into the hyaluronidase solution (300 μg/ml, Sigma) to disperse follicular cells. Follicular cells-free zygotes were washed and incubated in drops of M2 medium, under mineral oil (Sigma), at 37.5 °C, 5% CO 2 in the air until being used for microinjections [60] . Cocktail preparation and zygote injection Injection mixes were prepared on ice prior to use and were never frozen and used again. Microinjections were performed on zygotes 24–25 h post hCG, in a drop of M2 medium under mineral oil. Zygotes, were microinjected into the cytoplasm using Eppendorf 5242 microinjector (Eppendorf-Netheler-Hinz GmbH) and Eppendorf Femtotips II capillaries with the following CRISPR cocktail: Cas9 mRNA 25 ng/µl, sgRNA 15 ng/µl, and mFam46C_FLAG_oligo. Injected embryos were incubated in M2, in standard culture conditions for 30 min and next transferred into drops of M16 medium (Sigma) and cultured overnight. Embryo transfer After overnight culture microinjected embryos at 2-cell stage were transferred into the oviducts of 0.5-day p.c. pseudo-pregnant females. Usually, embryos were transferred into one oviduct only, and no more than 10–12 embryos into one female. Foster mothers were kept in individual cages until delivery of the pups. Four-weeks-old young were separated from foster mothers. Small fragments of their ears or tails were taken from anaesthetized animals to perform genotyping. Males and females from one foster mother were kept in separate cages. Mice genotyping Genomic DNA from ear or tail fragments was isolated and PCR was performed with Fam46C_seqF and Fam46C_seqR primer pair for detecting deletions of the catalytic domain and mF46cFLAG_seq1F, mF46cFLAG_seq1R primer pair for genotyping FLAG-tag insertions, DNA sequencing results were analyzed with Mutation Surveyor 4.0 software Demo (SoftGenetics). 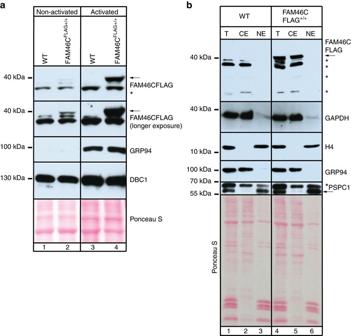Fig. 5 FAM46C is induced in activated B lymphocytes and localizes mainly in the cytosol.aSplenocytes fromFAM46C-FLAG +/+knock-in mice and control animals were isolated and then cultured in presence of IL4 and LPS for 72 h. The level of FAM46C-FLAG was checked by western blot in non-activated (lanes 1–2) and activated (lanes 2–4) cells. GRP94 was used as activation marker, while DBC1 was used as a loading control.bEndogenous FAM46C localizes mainly in the cytosol. Splenocytes from WT andFAM46C-FLAG+/+mice were isolated and fractionated. The whole-cell (T), cytoplasmic (CE), and nuclear (NE) extracts were analyzed by western blot. FAM46C-FLAG was detected using an anti-FLAG antibody. GAPDH and GRP94 were used as a cytosolic markers, while histone H4 and PSPC1 were used as nuclear markers.Arrowindicates the position of FAM46C-FLAG, whileasterisksindicts nonspecific bands detected by antibodies, which were present in samples isolated from both WT and FAM46C-FLAG animals FAM46C mice genotypes were shown in Supplementary Table 5 . Bone marrow analyses To determine bone marrow cellularity, the cells were counted on a Bürker hemocytometer and dead cells were excluded using trypan blue dye. To evaluate percentage of plasma cells bone marrow cells were blocked in 2% BSA for 15 min. 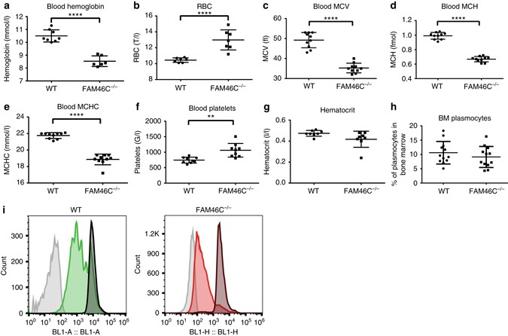Fig. 6 FAM46CKO 12-week-old mice display reduced blood hemoglobin levels and activated primary B lymphocytes proliferate faster.a–hHematologic parameters ofFAM46CKO and control animals:aBlood hemoglobin concentration (WT,n= 8;FAM46CKO,n= 6);bred blood cells count (RBC) (WT,n= 7;FAM46CKO,n= 7);cmean corpuscular volume (MCV) (WT,n= 10;FAM46CKO,n= 10);dmean corpuscular hemoglobin (MCH) (WT,n= 10;FAM46CKO,n= 10);emean corpuscular hemoglobin concentration (MCHC) (WT,n= 10;FAM46CKO,n= 10);fblood platelets (WT,n= 9;FAM46CKO,n= 9);gHematocrit (WT,n= 8;FAM46CKO,n= 8);hbone marrow (BM) plasmocytes (WT,n= 12;FAM46CKO,n= 12).P-values were calculated using two-way ANOVA tests (**P< 0.01, ****P< 0.0001).iAnalysis of the proliferation rate of activated primary B cells. B lymphocytes isolated fromFAM46CKO mice and matching WT controls were stained with CFSE and in vitro activated using IL4 and LPS. Cell divisions were monitored by levels of CFSE dilution. One representative experiment of 2 is presented. For each experiment splenic B lymphocytes from three individuals have been pulled, for both WT and mutant mice Next, the cells were labeled with anti-CD45.2 Horizon V500 (BD 562129) and anti-CD138-PE (BD 553714) monoclonal antibodies for 30 min at room temperature at 1:25 dilution, then washed with PBS and analyzed using LSR Fortessa and BD FACSDiva software version 8.0.1. The plasma cells were identified using CD138 from CD45.2-positive population. Discriminating positive vs. negative signals was ensured with fluorescence minus one (FMO) control. Blood analyses The blood samples were collected from 12-weeks-old WT and Fam46C KO mice of both sexes and were commercially analyzed at Veterinary Diagnostic Laboratory LabWet in Warsaw ( http://www.labwet.pl/ ) on the day of blood collection. Statistical analysis of the results was performed using GraphPad Prism6 software. Splenocytes fractionation Cell fractionation was performed using a REAP protocol [61] . Briefly, cells isolated from spleen of WT and FLAG-tagged knock-in mice were washed in ice-cold PBS then resuspended in ice-cold 0.1% NP40-PBS (Sigma) and centrifuged in benchtop microfuge at maximum speed for 10 s. Supernatant was collected as “cytosolic fraction” and remaining pellet was subsequently washed once with 0.1% NP40-PBS. Next nuclei pellet was resuspended in 0.1% NP40-0.5×PBS containing 500 U of viscolase (A&A Biotechnology), incubated at 37 °C for 30 min and designated as “nuclear fraction”. Collected fractions were supplemented with Laemmli sample buffer, separated in SDS-PAGE gels and analyzed with western blot approach. Data availability The RNA-seq data from this study have been submitted to the NCBI Gene Expression Omnibus (GEO; http://www.ncbi.nlm.nih.gov/geo/query/acc.cgi?acc=GSE83772 ) under accession number GSE83772. The mass spectrometry proteomics data have been deposited to the ProteomeXchange Consortium via the PRIDE partner repository with the dataset identifier PXD006790. All scripts used in bioinformatics analyses are available for researchers upon request. 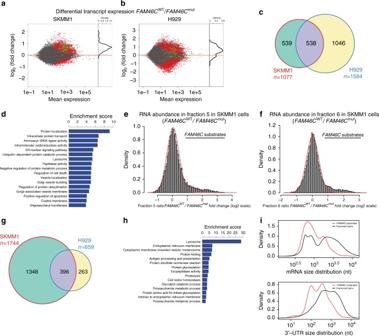Fig. 7 Global analysis of FAM46C substrates in MM cells.a,bMAplots of total RNA sequencing results representing differential expression analysis of FAM46CWT-GFP and FAM46Cmut-GFP-transduced MM cell lines. SKMM1 (a) and H929 (b) show transcriptome wide moderate deregulation of gene expression. Statistically significant values (FDR < 1%) are shown inred. The 396 transcripts constituting the common part for SKMM1 and H929 MM cell lines are marked withgreen circles.cVenn diagram demonstrating the overlap between upregulated transcripts in SKMM1 and H929 MM cell lines.dFunctional GO terms annotation clustering of significantly upregulated transcripts in both MM cell lines.e,fHistogram representing the distribution of FAM46C-dependent polyadenylation rations monitored in fraction #5 (e) and #6 (f) in SKMM1 cell lines. Modeled normal distribution is fitted as ared lineto emphasize the outlying population of FAM46C polyadenylated transcripts.gVenn diagram demonstrating the overlap between transcripts shifting to both long poly(A) fractions in FAM46WToverexpressing cells mutually in SKMM1 and H929 MM cell lines.h396 transcripts constituting the common part for SKMM1 and H929 MM cell lines were used in DAVID Functional Annotation Clustering Analysis.iThe same set of transcripts was used to characterize the 3′-UTRs and total mRNA lengths showing a bias towards shorter species in either 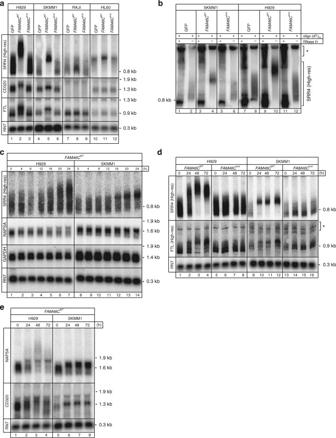Fig. 8 FAM46C expression results in polyadenylation of selected mRNAs in MM cells.aNorthern blot analysis ofSSR4,CD320, andFTLtranscripts from H929 (lanes 1–3), SKMM1 (lanes 4–6), Raji (lanes 7–9) and HL60 (lanes 10–12) cells transduced with GFP (lanes 1, 4, 7, 10), FAM46CWT-GFP (lanes 2, 5, 8, 11), and FAM46Cmut-GFP (lanes 3, 6, 9, 12).Asterisksindicate cross-hybridization signals.bTheSSR4transcript is extensively polyadenylated by FAM46C in MM cells. High-resolution northern blot analysis ofSSR4transcripts from SKMM1 (lanes 1–6) and H929 (lanes 7–12) transduced with GFP (lanes 1, 2, 7, 8), FAM46CWT-GFP (lanes 3, 4, 9, 10), and FAM46Cmut-GFP (lanes 5, 6, 11, 12) after RNase H treatment (lanes 1, 3, 5, 7, 9, 11) to remove the poly(A) tail in presence of oligo(dT)25. Control reactions were carried out in the presence of oligo(dT) without RNase H (lanes 2, 4, 6, 8, 10, 12). Kinetics of polyadenylation ofSSR4,NAPSA,FTL, andCD320transcripts over the time course ofFAM46Cexpression.cHigh- and low-resolution northern blot analysis ofSSR4,NAPSA,GAPDH, andRN7transcripts from H929 (lanes 1–7) and SKMM1 cells (lanes 8–14) transduced with FAM46CWT-GFP up to 24 h.dHigh-resolution northern blot analysis ofSSR4andFTLtranscripts from H929 (lanes 1–8) and SKMM1 cells (lanes 9–16) transduced with FAM46CWT-GFP (lanes 1–4, 9–12) and FAM46Cmut-GFP (lanes 5–8, 13–16) up to 72 h.eNorthern blot analysis ofNAPSAandCD320transcripts from H929 (lanes 1–4) and SKMM1 cells (lanes 5–8) transduced with FAM46CWT-GFP up to 72 h 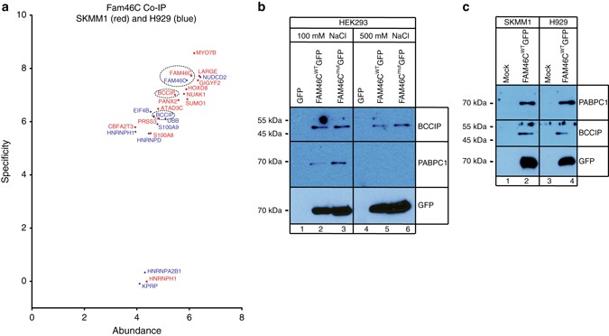Fig. 9 FAM46C interacts with BCCIPβ and PABPC1 in human cells.aVisualizations of Co-IP-MS experiments using GFP-tagged FAM46C expressed in myeloma cells H929 (shown inblue) and SKMM1 (shown inred). Estimated quantities of identified proteins were calculated using the label-free quantification (LFQ) algorithm and are represented as dot–plot graphs. Protein abundance was calculated as LFQ intensity of the protein signal divided by its molecular weight and is shown on thexaxis on a logarithmic scale. Specificity was defined as the ratio of protein LFQ intensity measured in the bait Co-IP to the background level (protein LFQ intensity in a sample) and is shown on theyaxis on a logarithmic scale.b,cWestern-blot detection of BCCIPβ and PABPC1 co-immunoprecipitated with:bFAM46CWT-GFP and FAM46Cmut-GFP from stable HEK293 cell lines;cFAM46CWT-GFP from transduced SKMM1 and H929 MM cell lines. Purification was performed at low (lanes 1–3) and high (lanes 4–6) ionic strengths. GFP-tagged FAM46C was detected with α-GFP antibodies. Please note that the lack of the GFP signal in the GFP only control (lanes 1 and 4) is because the blot was cutoff to avoid very strong GFP signal, which could influence the readout All other remaining data are available within the Article and Supplementary Files or available from the authors upon request.